Truly work-like work extraction via a single-shot analysis The work content of non-equilibrium systems in relation to a heat bath is often analysed in terms of expectation values of an underlying random work variable. However, when optimizing the expectation value of the extracted work, the resulting extraction process is subject to intrinsic fluctuations, uniquely determined by the Hamiltonian and the initial distribution of the system. These fluctuations can be of the same order as the expected work content per se , in which case the extracted energy is unpredictable, thus intuitively more heat-like than work-like. This raises the question of the ‘truly’ work-like energy that can be extracted. Here we consider an alternative that corresponds to an essentially fluctuation-free extraction. We show that this quantity can be expressed in terms of a one-shot relative entropy measure introduced in information theory. This suggests that the relations between information theory and statistical mechanics, as illustrated by concepts like Maxwell’s demon, Szilard engines and Landauer’s principle, extends to the single-shot regime. The amount of useful energy that can be harvested from non-equilibrium systems not only characterizes practical energy extraction and storage, but is also a fundamental thermodynamic quantity. Intuitively, we wish to extract ordered and predictable energy, that is, ‘work’, as opposed to disordered random energy in the form of ‘heat’. The catch is that, in statistical systems, the work cost or yield of a given transformation is typically a random variable [1] . As an example, one can think of the friction that an object experiences when forced through a viscous medium. On a microscopic level, this force resolves into chaotic molecular collisions and thus results in a random work cost each time we perform this transformation. This is further illustrated by experimental tests [2] , [3] , [4] of ‘fluctuation theorems’, which characterize the randomness in the work cost (or ‘entropy production’) of non-equilibrium processes [1] . These observations raise the question of a quantitative notion of work content that truly reflects the idea of work as ordered energy. Here, we show that standard expressions for the work content [5] , [6] , [7] , [8] can correspond to a very noisy and thus heat-like energy, but we also introduce an alternative that quantifies the amount of ordered energy that can be extracted. The latter can be expressed in terms of a non-equilibrium generalization of the free energy, or equivalently in terms of a one-shot information-theoretic relative entropy, which quantifies how ‘far’ the given non-equilibrium system is from thermal equilibrium. ‘Standard’ information theory typically quantifies the resources needed to perform a given information-theoretic task averaged over many repetitions, for example, the average number of bits needed to send many independent messages [9] . In contrast, ‘one-shot’ (or ‘single-shot’) information theory rather focuses on single instances of such tasks (see, for example, refs 10 , 11 ). Given the strong historical links between standard information theory and the work extraction problem, via concepts like Szilard engines, Landauer’s principle and Maxwell’s demon [12] , [13] , it is reasonable to ask whether also one-shot information theory has a counterpart in statistical mechanics. Together with refs 14 , 15 , 16 , 17 , 18 , 19 , the results of this investigation suggest that this is indeed the case. A direct consequence of the present investigation is that the results of refs 14 , 15 , 19 is brought into a more physical setting, allowing, for example, systems with non-trivial Hamiltonians, proof of near-optimality, as well as a connection to fluctuation theorems [1] . The latter suggests that the effects we consider become relevant in the typical regimes of fluctuation theorems. Similar results as in this study have been obtained independently in ref. 16 . See also recent results in ref. 17 based on ideas in ref. 18 . (For further discussions on the relations to the existing literature, see Supplementary Note 1 .) Work extraction The amount of work that a system can perform while it equilibrates with respect to an environment of temperature T is often [5] , [6] , [7] , [8] expressed as Here q is the state of the system, G ( h ) its equilibrium state, h the system Hamiltonian and k Boltzmann’s constant. For the simple model we employ here, q is a probability distribution over a finite set of energy levels, and D ( q || p )=∑ n q n log 2 q n −∑ n q n log 2 p n is the relative Shannon entropy (Kullback–Leibler divergence) [9] , and log 2 denotes the base 2 logarithm. The quantity ( q , h ), and the closely related cost of information erasure (Landauer’s principle), is often understood as an expectation value of an underlying random work yield (see, for example, refs 5 , 7 , 20 , 21 ). However, this tells us very little about the fluctuations, and thus the ‘quality’ of the extracted energy. Here, we show that optimizing the expected gain leads to intrinsic fluctuations. These can be of the same order as the expected work content ( q , h ) per se , in which case the work extraction does not act as a truly ordered energy source. As an alternative, we introduce the ɛ -deterministic work content, which quantifies the maximal amount of energy that can be extracted if we demand to always get precisely this energy each single time we run the extraction process, apart from a small probability of failure ɛ . Hence, in contrast to the expected work extraction, where we do not put any restrictions on how broadly distributed the random energy gain is, we do in the ɛ -deterministic work extraction demand that the probability distribution should be very peaked, that is, very predictable. In other words, the ɛ -deterministic work content formalizes the idea of an almost perfectly ordered energy source. The model Our analysis is based on a very simple model of a system interacting with a heat bath of fixed temperature T (see Fig. 1 ). Akin to, for example, refs 15 , 21 , 22 , we model the Hamiltonian of the system as finite set of energy levels h =( h 1 ,…, h N ). The state of the system we regard as a random variable , with a probability distribution q =( q 1 ,…, q N ). On this system, we have two elementary operations. 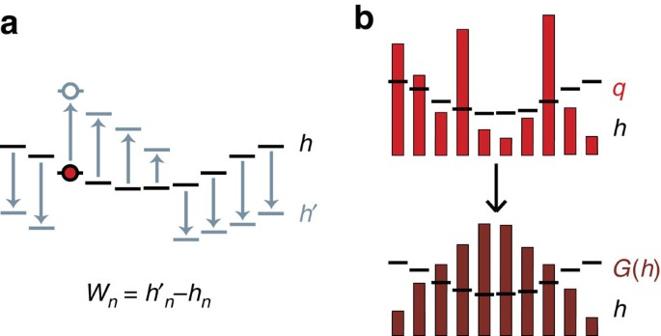Figure 1: The model. The system can be in any of the states 1,…,N, each assigned an energy level (horizontal lines)h=(h1,…,hN). Two elementary operations modify the system: (a) LT. This lifts or lowers the energy levelshto a new configurationh′, but leaves the state (circle) intact. If the system is in staten, the work cost of the LT is defined as. (b) Thermalization with respect to a heat bath of temperatureT. This changes the initial probability distribution (bars)q=(q1,…,qN) over the states, into the Gibbs distributionG(h), but leaves the energy levelshintact, and has no work cost. We build up processes by combining LTs and thermalizations. Figure 1: The model. The system can be in any of the states 1,…, N , each assigned an energy level (horizontal lines) h =( h 1 ,…, h N ). Two elementary operations modify the system: ( a ) LT. This lifts or lowers the energy levels h to a new configuration h ′, but leaves the state (circle) intact. If the system is in state n , the work cost of the LT is defined as . ( b ) Thermalization with respect to a heat bath of temperature T . This changes the initial probability distribution (bars) q= ( q 1 ,…,q N ) over the states, into the Gibbs distribution G ( h ), but leaves the energy levels h intact, and has no work cost. We build up processes by combining LTs and thermalizations. Full size image The first of these two operations changes the energy levels h to a new set of energy levels h ′, but leaves the state, and thus the probability distribution q , intact. We refer to this as level transformations (LTs). (For a quantum system, this would essentially correspond to adiabatic evolution with respect to some external control parameters, that is, in the limit of infinitely slow changes of the control we alter the energy levels, but not how they are occupied.) Via the LTs we define what ‘work’ is in our model. If we perform an LT that changes h to h ′, and if the system is in state n , then this results in a work gain (or work cost ). As the work gain depends on the state of the system, a random state implies a random work gain. The second elementary operation corresponds to thermalization, where one can imagine that we connect the system to the heat bath, let it thermalize and slowly de-connect it again. We model this by putting the system into the random state described by the Gibbs distribution, P ( = n )= G n ( h ), where , β =1/( kT ) and is the partition function. It is furthermore assumed that the state (regarded as a random variable) after a thermalization is independent of the state before. We construct processes by combining these two types of elementary operations into any sequence of our choice. The resulting work yield of the process is defined as the sum of the work yields of all the LTs. (For a more detailed description of the model, see Supplementary Note 2 .) An example is given in Fig. 2 , where we construct the analogue of isothermal reversible (ITR) processes, which serve as a building block in our analysis (see Supplementary Note 3 ). As opposed to other processes we will consider, the ITRs have essentially fluctuation-free work costs. 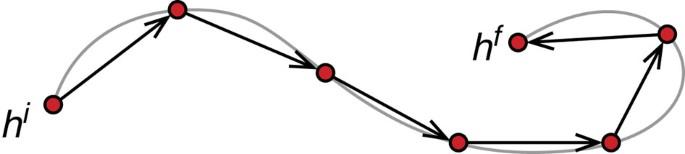Figure 2: ITR processes. In the space of energy level configurations, we connect an initial configurationhi∈Nwith the finalhf∈Nby a smooth path (grey line). Given anL-step discretization of this path, we construct a sequence of LTs (arrows) sandwiched by thermalizations (circles). This process has the random work cost, wherelis the state at thel-th step, which is Gibbs distributed G(hl). In the limit of an infinitely fine discretization, the expected work cost is limL→∞〈W〉=F(hf)−F(hi). The independence of the work costs of the subsequent LTs yields limL→∞(〈W2〉−〈W〉2)=0, that is, the work cost is essentially deterministic. Figure 2: ITR processes. In the space of energy level configurations, we connect an initial configuration h i ∈ N with the final h f ∈ N by a smooth path (grey line). Given an L -step discretization of this path, we construct a sequence of LTs (arrows) sandwiched by thermalizations (circles). This process has the random work cost , where l is the state at the l -th step, which is Gibbs distributed G( h l ). In the limit of an infinitely fine discretization, the expected work cost is lim L →∞ 〈 W 〉= F ( h f )− F ( h i ). The independence of the work costs of the subsequent LTs yields lim L →∞ (〈 W 2 〉−〈 W 〉 2 )=0, that is, the work cost is essentially deterministic. Full size image Expected work extraction Given an initial state with distribution q , we can reproduce equation (1) within our model. A cyclic three-step process, as described in Fig. 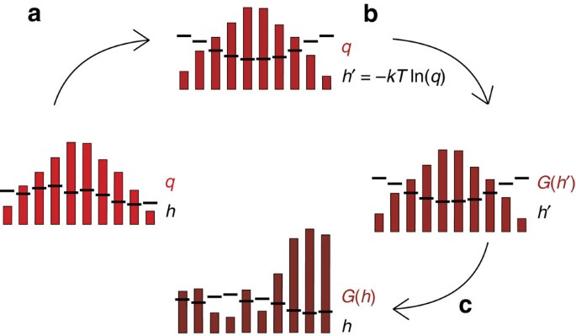Figure 3: Expected work extraction. For an initial statewith distributionq(bars) and energy levelsh(horizontal lines), the expected work content(q,h) is obtained by a cyclic three-step process. The idea is to avoid unnecessary dissipation when the system is put in contact with the heat bath. To this end, we make an LT to a set of energy levelsh′ for whichG(h′)=q. The total process is: (a) LT that transformshninto. (b) Thermalization, resulting in the Gibbs distributionG(h′)=q. (c) ITR process fromh′ back toh. The resulting random work yield is, with expectation value 〈Wyield〉=kTln(2)D(q||G(h)). 3 , gives the random work yield Figure 3: Expected work extraction. For an initial state with distribution q (bars) and energy levels h (horizontal lines), the expected work content ( q , h ) is obtained by a cyclic three-step process. The idea is to avoid unnecessary dissipation when the system is put in contact with the heat bath. To this end, we make an LT to a set of energy levels h ′ for which G ( h ′)= q . The total process is: ( a ) LT that transforms h n into . ( b ) Thermalization, resulting in the Gibbs distribution G ( h ′)= q . ( c ) ITR process from h ′ back to h . The resulting random work yield is , with expectation value 〈 W yield 〉= kT ln(2) D ( q || G ( h )). Full size image By taking the expectation value, we obtain equation (1). The positivity of relative entropy, D ( q || p )≥0, can be used to show that no process can give a better expected work yield ( Supplementary Note 4 ). One can in a similar fashion determine the minimal expected work cost for information erasure (see Supplementary Note 5 ). Fluctuations in expected work extraction How large are the fluctuations for a process that maximizes the expected work extraction, and thus achieves ( q , h )? Equation (2) determines the noise of the specific process in Fig. 3 , but it turns out that it actually specifies the fluctuations for all processes that optimize the expected work extraction. (For the exact statement, see Methods, or Supplementary Note 6 .) We can conclude that to analyse the noise in the optimal expected work extraction, it is enough to consider equation (2). As we will confirm later, these fluctuations can be of the same order as ( q , h ) itself. ɛ -deterministic work extraction As the optimal expected work extraction suffers from fluctuations, a natural question is how much (essentially) noise-free energy can be extracted. We say that a random variable X has the ( ɛ , δ )-deterministic value x , if the probability to find X in the interval [ x − δ , x + δ ] is larger than 1− ɛ . Hence, δ is the precision by which the value x is taken, and ɛ the largest probability by which this fails. (See Supplementary Note 7 for further properties.) We define as the highest possible ( ɛ, δ )-deterministic work yield among all processes that operate on the initial distribution q with initial and final energy levels h . Next, we define the ɛ -deterministic work content as , that is, we take the limit of infinite precision, thus formalizing the idea of an energy extraction that is essentially free from fluctuations. ɛ ( q, h ) can be expressed in terms of the ɛ -free energy, which is defined via restrictions to sufficiently likely subsets of energy levels. Given a subset Λ, we define . We minimize Z Λ ( h ) among all subsets Λ such that q (Λ)=∑ n ∈ Λ q n >1− ɛ . If Λ * is such a minimizing set, then the ɛ -free energy is defined as F ɛ ( q,h )=− kT ln Z Λ* ( h ). (See Supplementary Note 8 for further explanations.) The concept of one-shot free energy has been introduced independently in ref. 16 . The distribution of fluctuations is clearly important for determining the value of ɛ ( q, h ). It is thus maybe not surprising that a variation (see Methods) of Crook’s fluctuation theorem [23] can be used to prove where ‘≈’ signifies that the equality is true up to a small error (see Methods, or Supplementary Note 9 and Supplementary Note 10 ). The error is small in the sense that it can be regarded as the energy of a sufficiently likely equilibrium fluctuation (see Methods and Supplementary Note 11 ). An example of a process that gives the right-hand side of equation (3) is described in Fig. 4. In the case of completely degenerate energy levels h =( r ,…, r ), equation (3) reduces to the result in ref. 14 . (See also Supplementary Note 12 and Supplementary Note 13 for the ɛ -deterministic cost of information erasure). The above result can be reformulated in terms of an ɛ -smoothed relative Rényi 0-entropy, defined as This relative entropy was (up to some technical differences) introduced in ref. 24 in the context of one-shot information theory. (See refs 25 , 26 for quantum versions.) One can see that Comparisons An immediate question is how ( q, h ) compares with ɛ ( q, h ), and with the fluctuations in the optimal expected work extraction. The latter we measure by the s.d. of W yield in equation (2), . We compare how these three quantities scale with increasing system size (for example, in number of spins, or other units). Our first example is a collection of m systems whose state distributions are independent and identical, q m ( n 1 ,…, n m )= q ( n 1 )… q ( n m ), and which have non-interacting identical Hamiltonians, corresponding to energy levels h m ( n 1 ,…, n m )= h ( n 1 )+…+ h ( n m ). In this case ( q m , h m )= m ( q , h ), and , where σ ( q || r ) 2 =∑ n q n [log 2 ( q n / r n )] 2 − D ( q || r ) 2 . By Berry–Esseen’s theorem [27] , [28] (see Methods and Supplementary Note 14 ), one can show that ɛ ( q m , h m ) is equal to m ( q, h ) to the leading order in m (see ref. 29 for a similar result in a resource theory framework). The difference only appears at the next to leading order. Hence, in these systems the fluctuations are comparably small, and the dominant contribution to ɛ ( q m , h m ) is ( q m , h m ). It appears reasonable to expect similar results for non-equilibrium systems with sufficiently fast spatial decay of both correlations and interactions, which may explain why issues concerning as a measure of work content appear to have gone largely unnoticed. A simple modification of the state distribution in the previous example results in a system with large fluctuations. With probability 1− ɛ (independent of m ), the system is prepared in the joint ground state 0,…, 0, and with probability ɛ in the Gibbs distribution. This results in and yields ( q m , h m ) ∼ − mkT ln(2)(1− ɛ )log 2 G 0 ( h ), and ɛ ( q m , h m ) ∼ − mkT ln(2)log 2 G 0 ( h ). Hence, all three quantities grow proportionally to m . For a second case of large fluctuations, we choose the distribution , for a collection of d -level systems. For large m , we assume that the energy levels are dense enough that they can be replaced by a spectral density. One example is Wigner’s semicircle law, where for | x |≤ R ( m ). With , this is the asymptotic energy level distribution of large random matrices from the Gaussian unitary ensemble [30] . For the semicircle distribution ( q m , h m ) ∼ R ( m ), , and ɛ ( q m , h m ) ∼ c ( ɛ ) R ( m ), where c ( ɛ ) is independent of m . We have here employed what one could refer to as a discrete classical model. Relevant extensions include a classical phase-space picture, as well as a quantum setting that allows superpositions between different energy eigenstates (for example, in the spirit of refs 16 , 29 , 31 ) and where the work-extractor can possess quantum information about the system [15] . An operational approach, based on what ‘work’ is supposed to achieve, rather than ad hoc definitions, may yield deeper insights to the question of the truly work-like energy content. It is certainly justified to ask for the relevance of the effects we have considered here. The evident role of fluctuations suggests that the noise in the expected work extraction should become noticeable in the same nano-regimes as where fluctuation theorems are relevant. The considerable experimental progress on the latter (see, for example, refs 2 , 3 , 4 ) should reasonably be applicable also to the former. Also the theoretical aspects of the link to fluctuation theorems merits further investigations. We have seen that the ɛ -deterministic work content to the leading order becomes equal to the expected work content for systems with identical non-interacting Hamiltonians and identical uncorrelated state distributions. However, we have also demonstrated by simple examples that the expected work extraction can become very noisy when we deviate from this simple setup. In these cases, the expected work extraction thus fails to capture our intuitive notion of work as ordered energy, while the ɛ -deterministic work extraction is predictable by construction. One might object that many realistic systems are approximately non-interacting and approximately uncorrelated, and thus presumably show no significant difference between the ɛ -deterministic and the expected work extraction. However, as we here consider a general non-equilibrium setting, there is no particular reason to assume, for example, weak correlations. It is maybe also worth to point out that the fluctuations in the expected work extraction can be large also outside the microscopic regime, as this only requires a sufficiently ‘violent’ relation between the non-equilibrium state and the Hamiltonian of the system. As opposed to the expected work content, the ɛ -deterministic work content retains its interpretation as the ordered energy. It is no coincidence that this is much analogous to how single-shot information theory generalizes standard information theory [10] , [11] . In this spirit, the present study, along with refs 14 , 15 , 16 , 17 , 18 , 19 , can be viewed as the first glimpse of a ‘single-shot statistical mechanics’. Randomness in optimal expected work extraction In the main text, we briefly mentioned the fact that processes that optimize the expected work extraction converge to the random variable in equation (2). We can phrase this result more precisely as follows. For a process that operates on an initial state with distribution q , we let W yield ( , ) denote the corresponding random work yield. We here consider cyclic processes that starts and ends in the energy levels h . If is a family of processes such that lim m→∞ 〈 W yield ( m , )〉= ( q , h ), then in probability. (For a proof see Supplementary Note 6 ). Bounds on the ɛ -deterministic work content The exact statement of equation (3) is In Supplementary Note 11 , it is shown that − kT ln(1− ɛ ) is an upper bound to the ɛ -deterministic work content of equilibrium systems. Equation (5) thus determines the value of ɛ ( q , h ) up to an error with the size of a sufficiently probable equilibrium fluctuation. We obtain the lower bound in equation (5) by the process described in Fig. 4 . The upper bound is obtained by a combination of a variation ( Supplementary Note 10 , Supplementary Equation (S73) ) on Crook’s fluctuation theorem [23] and a work bound for LTs ( Supplementary Note 10 ). For a discussion on an alternative single-shot work extraction quantity, and its relation to ɛ , see Supplementary Note 15 . 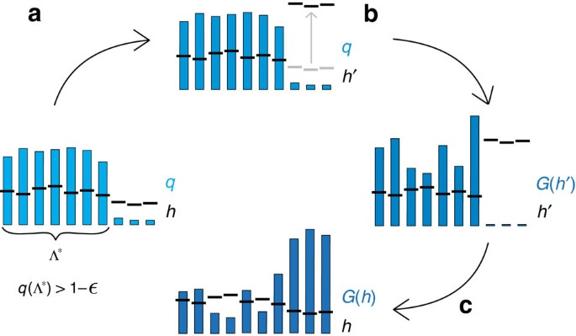Figure 4:ɛ-deterministic work extraction. For a state distributionqand energy levelsh, let Λ*be a subset of the energy levels such thatFɛ(q,h)=−kTlnZΛ*(h). (a) LT that lifts all energy levels not in Λ*to a very high value, that is,ifn∈Λ*, whileifn∉Λ*. (b) Thermalization, resulting in the Gibbs distributionG(h′). (c) ITR process fromh′ back toh, which gives the essentially deterministic work yieldF(h′)−F(h). In the limitE→+∞, this process gives the work yieldFɛ(q,h)−F(h) with a probability larger than 1−ɛ. This is a lower bound toɛ(q,h), but is also close to it for smallɛ. Figure 4: ɛ -deterministic work extraction. For a state distribution q and energy levels h , let Λ * be a subset of the energy levels such that F ɛ ( q , h )=− kT ln Z Λ* ( h ). ( a ) LT that lifts all energy levels not in Λ * to a very high value, that is, if n ∈ Λ * , while if n ∉ Λ * . ( b ) Thermalization, resulting in the Gibbs distribution G ( h ′). ( c ) ITR process from h ′ back to h , which gives the essentially deterministic work yield F ( h ′)− F ( h ). In the limit E →+∞, this process gives the work yield F ɛ ( q , h )− F ( h ) with a probability larger than 1− ɛ . This is a lower bound to ɛ ( q , h ), but is also close to it for small ɛ . Full size image Expansion of ɛ in the multi-copy case In the case of a state distribution q m ( n 1 ,…, n m )= q ( n 1 )… q ( n m ), and energy levels h m ( n 1 ,…, n m )= h ( n 1 )+…+ h ( n m ), the ɛ -deterministic work content has the expansion where is a correction term that grows slower than , and Φ −1 is the inverse of the cumulative distribution function of the standard normal distribution. The smaller our error tolerance ɛ , the more the correction term lowers the value of ɛ ( q m , h m ) as compared with ( q m , h m ). This expansion is proved via Berry–Esseen’s theorem [27] , [28] , which determines the convergence rate in the central limit theorem (see Supplementary Note 14 ). How to cite this article: Åberg J. Truly work-like work extraction. Nat. Commun. 4:1925 doi: 10.1038/ncomms2712 (2013).